Single-shot ultrafast tomographic imaging by spectral multiplexing Computed tomography has profoundly impacted science, medicine and technology by using projection measurements scanned over multiple angles to permit cross-sectional imaging of an object. The application of computed tomography to moving or dynamically varying objects, however, has been limited by the temporal resolution of the technique, which is set by the time required to complete the scan. For objects that vary on ultrafast timescales, traditional scanning methods are not an option. Here we present a non-scanning method capable of resolving structure on femtosecond timescales by using spectral multiplexing of a single laser beam to perform tomographic imaging over a continuous range of angles simultaneously. We use this technique to demonstrate the first single-shot ultrafast computed tomography reconstructions and obtain previously inaccessible structure and position information for laser-induced plasma filaments. This development enables real-time tomographic imaging for ultrafast science, and offers a potential solution to the challenging problem of imaging through scattering surfaces. In 1968, when computed tomography (CT) was conceived, the initial scans required several days to complete and the reconstructions were plagued by errors caused by changes in the subject, as it moved or decomposed [1] . Since then, there has been a constant push to increase the speed of tomographic imaging in order to reduce movement artifacts and allow characterization of dynamically varying objects. Today, the fastest medical scanners, designed for cardiac imaging, can run at about 10 frames per second (fps), limited by the mechanical factors associated with a rotating source and detector [2] . Non-medical systems have achieved rates up to 10,000 fps by using fixed detectors and scanning the source non-mechanically, enabling visualization of dynamic flows and beating hearts of small, live animals [3] . Tomographic imaging of ultrafast phenomena has remained problematic, however, as required temporal resolutions in the picosecond and femtosecond range cannot be achieved by traditional scanning methods. Although ultrafast resolution has been achieved on a multi-shot basis by using short-pulse optical techniques and rotating the object [4] , this approach will not work for a large class of phenomena that vary from shot to shot, requiring the use of single-shot probing methods. [5] , [6] Recently, Li et al . [7] have made progress in this direction by demonstrating simultaneous acquisition of four projections using separate single-shot probe lines. Sparse angle-sampling, however, is well known to result in artifacts that can strongly affect the reconstructed images [8] . Here we introduce a technique, spectrally multiplexed tomography (SMT), which provides single-shot, ultrafast CT imaging with a continuous range of angles. In the SMT concept, multiplexing, which is the key to single-shot CT, is done spectrally. The wavelength of a broadband source is used to encode the position of rays probing the object (or alternatively the angle), allowing projection measurements taken from different angles simultaneously to be distinguished. We apply SMT to measure two-dimensional (2D) cross-sectional electron-density profiles of laser-induced plasma (LIP) filaments with high precision. Characterization of these profiles is of critical importance to many applications involving laser–plasma interactions, such as laser–plasma accelerators, where the plasma density and the formation of plasma filaments plays an important role in determining the performance and stability [9] , [10] . Traditional diagnostics, which probe the plasma from a single direction, require the assumption of a single filament with axial symmetry to allow reconstruction of the density distribution [11] , resulting in errors for non-symmetric or heterogeneous profiles. Tomographic probing, by contrast, can resolve arbitrarily shaped plasmas, improving the density measurement and allowing for the presence of multiple, asymmetric filaments. We demonstrate the capability to detect the presence and position of two plasma filaments positioned so that they would be indistinguishable using the traditional single-projection approach, and show that we can resolve the ellipticity of an individual filament cross-section. SMT of a point-like plasma target Spectral multiplexing using position encoding was implemented by focusing a spectrally broadband laser with angular dispersion, resulting in a linearly distributed array of spectrally distinct fan-beam sources ( Fig. 1a ). The angular extent of each source, set by the focusing geometry, was 12°, and the transverse position of each focus, x in , was correlated linearly to its wavelength. An imaging spectrometer was used to resolve the transverse position ( x out ) and wavelength ( λ ) of each ray at a plane (S out ) two millimetres downstream of the focal plane (S in ). The entrance slit of the spectrometer was used to select a subset of the rays, defining a measurement plane perpendicular to the plasma filaments ( Fig. 1b ). Frequency-domain interferometry [12] was then used to measure the phase shift experienced by each ray, resulting in a phase image, Φ ( x in , x out ) where each point corresponded to a unique trajectory through the interaction. 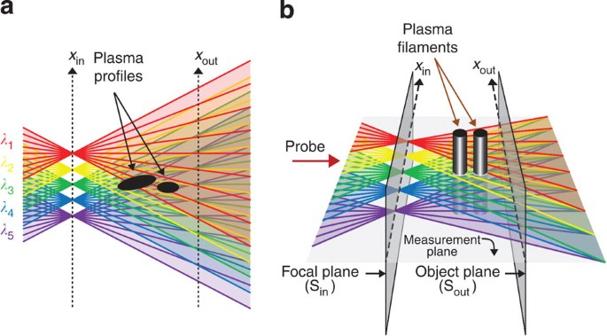Figure 1: Position-encoded implementation of spectral multiplexing. (a), Array of fan beam sources with distinct wavelengths, {λ1, ...λ5} and foci distributed alongxin. Although the diagram depicts discretely distributed sources for clarity, the wavelength (and thus source) dispersion is continuous. The plasma cross-sectional profiles are shown as black ovals. (b), 3D perspective drawing showing the orientation of the focal plane, Sin, the object plane, Sout, and the measurement plane relative to the fan beam sources and the plasma filaments. Two plasma filaments aligned perpendicular to the measurement plane were separated along the direction of probe propagation. Figure 1: Position-encoded implementation of spectral multiplexing. ( a ), Array of fan beam sources with distinct wavelengths, { λ 1 , ... λ 5 } and foci distributed along x in . Although the diagram depicts discretely distributed sources for clarity, the wavelength (and thus source) dispersion is continuous. The plasma cross-sectional profiles are shown as black ovals. ( b ), 3D perspective drawing showing the orientation of the focal plane, S in , the object plane, S out , and the measurement plane relative to the fan beam sources and the plasma filaments. Two plasma filaments aligned perpendicular to the measurement plane were separated along the direction of probe propagation. 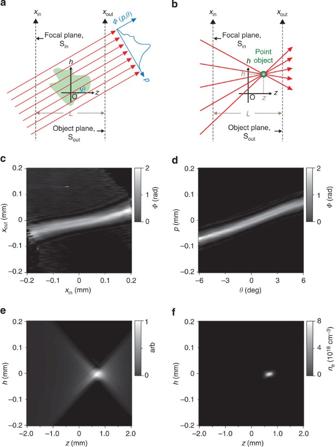Figure 2: Tomographic measurement of the cross-sectional profile of a laser-induced plasma filament. (a) Schematic showing the relationship between the phase image coordinates (xin,xout), the sinogram coordinates (p,θ) and the electron-density coordinates (z,h). (b) Schematic illustrating the relationship defined betweenxinandxoutfor a point located at (z,h). (c) Phase image for a single laser-induced plasma. (d) Sinogram resulting from the interpolation of the data incfrom the (xin,xout) to the (p,θ) coordinate system. (e) Back-projection generated from sinogram ind. (f) Reconstructed electron-density after deconvolution of the back-projection inewith the PSF. Full size image Figure 2 depicts the SMT reconstruction procedure for a sample LIP composed of a single filament. The phase image ( Fig. 2c ) is characterized by an angled band of nearly uniform width and phase shift. The angle can be understood by considering the contribution to the phase image from an infinitesimal point-object in the ( z , h ) density space ( Fig. 2b ). Each ray intersecting this point accrues the same amount of phase shift, determined by the density at that point, and the set of all such rays defines a linear relationship between the input and output coordinates: Figure 2: Tomographic measurement of the cross-sectional profile of a laser-induced plasma filament. ( a ) Schematic showing the relationship between the phase image coordinates ( x in , x out ), the sinogram coordinates ( p , θ ) and the electron-density coordinates ( z , h ). ( b ) Schematic illustrating the relationship defined between x in and x out for a point located at ( z , h ). ( c ) Phase image for a single laser-induced plasma. ( d ) Sinogram resulting from the interpolation of the data in c from the ( x in , x out ) to the ( p , θ ) coordinate system. ( e ) Back-projection generated from sinogram in d . ( f ) Reconstructed electron-density after deconvolution of the back-projection in e with the PSF. Full size image The locus of equation (1) within the phase image is a line of uniform phase with slope, m , determined by the longitudinal position of the point, and intercept, b , determined by the transverse position. An arbitrary object can be thought of as a sum of such points, each contributing distinct lines of phase. For the case of a phase band as in Fig. 2c , a highly localized object is implied, with transverse size determined by the width of the band, and longitudinal position by its angle, α , given by α ( z )=tan −1 m ( z ). The reconstruction of the plasma-density profile was done by a process of back-projection [8] and deconvolution. To implement the back-projection, the phase image was first re-sampled onto the projection coordinates, ( p , θ ), yielding a 'sinogram' ( Fig. 2d ), which represents the information that would be obtained by a series of parallel-projection beams as a function of angle. The back-projection ( Fig. 2e ) resulting from this sinogram has a characteristic bow–tie shape due to the lack of complete angular coverage in the sinogram. This shape, which is intrinsic to the geometry of the detection setup, can be modelled as the effect of a point-spread function (PSF) relating the electron-density space to the back-projection space. The PSF was estimated by applying the back-projection algorithm to a function of the form: which approximates a 2D Dirac-Delta function for sufficiently small Δ r . Here, we used Δ r= 1 μm, as this value was significantly smaller than the spatial resolution of the imaging system. The cross-sectional electron-density profile ( Fig. 2f ) was then recovered by performing a 2D deconvolution of the back-projection image with the PSF. The resulting density profile is clean and free of the bow–tie feature. The quality of the reconstruction is surprisingly high, given the small range of probing angles. This result is attributable, in part, to the fact that the angle-sampling is essentially continuous and may be counted as one of the benefits of SMT. A scaling argument may be used to show (in the case of continuous angle-sampling over a limited angular range) that measurement of an object with a small range of angles is mathematically equivalent to the measurement of a longitudinally scaled-up copy of the object using a larger range of angles. This statement is equivalent to saying that the primary effect of limiting the range of angles, in this case, is the loss of longitudinal resolution, rather than the generation of artifacts. Depth perception The principal benefit of tomography is the ability to resolve both the depth of a feature and its longitudinal structure, where longitudinal refers to the direction of probing. To test the depth perception of SMT, tomographic images of the LIP were taken as it was scanned longitudinally over a range of 2.4 mm between S in and S out . The measured and expected positions were then compared using an analysis of both the phase-band angles ( Fig. 3a ) and the reconstructed density profiles ( Fig. 3b ). 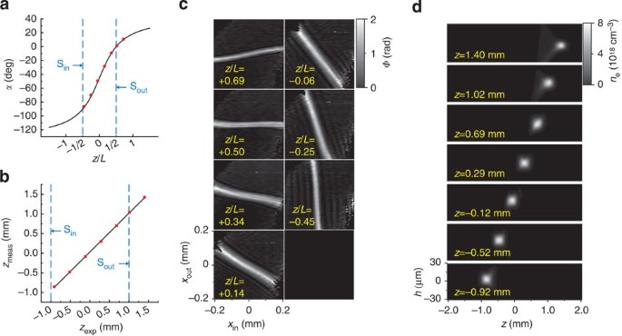Figure 3: Longitudinal position sensitivity of SMT. (a) Comparison of the measured angle (red dots) and predicted angle (black curve) of the phase band versus normalized longitudinal positionz/L. (b) Plot of the measured longitudinal position,zMeas, determined from the tomographic reconstruction (red squares) versus the expected position,zExp, determined from the micrometer on the scan stage. A linear-fit to the data (black line) has a slope of 0.986. (c) Phase images at each scan position. (d) Reconstructed electron-density profiles at each scan position. Figure 3: Longitudinal position sensitivity of SMT. ( a ) Comparison of the measured angle (red dots) and predicted angle (black curve) of the phase band versus normalized longitudinal position z / L . ( b ) Plot of the measured longitudinal position, z Meas , determined from the tomographic reconstruction (red squares) versus the expected position, z Exp , determined from the micrometer on the scan stage. A linear-fit to the data (black line) has a slope of 0.986. ( c ) Phase images at each scan position. ( d ) Reconstructed electron-density profiles at each scan position. Full size image Figure 3c shows phase images for each position of the scan. The angle of the phase band clearly changes with longitudinal position, as prescribed by equations (1–3). From equation (2), it is evident that the rotation of the phase band scales with the distance between the focal and object planes, L , allowing for an intuitive interpretation of the rotation. When z / L = −1/2, the plasma is located at S in , and the angle, α =−90°, corresponds to a vertical band ( Fig. 3c ). As S in corresponds to the focal plane, a point located there is probed by a single source of a single wavelength (that is, one input position, x in ) and the phase shadow is projected onto all output positions, x out . When z / L = +1/2, the plasma is located at S out and α =0 ° corresponds to a horizontal band. In this case, the point is probed by many sources (that is, many wavelengths and many x in ), but casts a phase shadow at only one x out . The excellent agreement between measurement and theory, shown in Fig. 3a , indicates that the ray picture of probe propagation presented above is valid. Although the full region between lenses L1 and L2 is probed, the region between S in and S out is where the phase-band angle is the most sensitive to changes in z / L . As z / L = +1/2 also corresponds to the plane that is imaged onto the spectrometer detector, this location presents itself as the optimal one for SMT. A comparison was also done between the centroid position of the reconstructed plasma profiles (shown in Fig. 3d ) and the expected position derived from the indicator of the micrometre actuator used to control the position of the plasma. A linear best fit to the data was done, and the slope was found to be 0.986, indicating an error of <2%, and thus a deviation of <32 μm over the full range of the scan. The recovered electron-density profiles did not change significantly over the range of the scan, providing confidence that the reconstructions were reasonable. Resolving multiple filaments To test SMT's ability to resolve longitudinal structure, a two-filament plasma target was created by combining two pump lasers with a small angle onto a single off-axis parabolic mirror (see Methods). The resulting laser-induced filaments overlapped transversely, but were separated longitudinally, as shown in Fig. 1b . In this configuration, the traditional diagnostic, which is equivalent to a measurement using only the θ =0 projection of SMT, would not be able to resolve the presence of a second filament. This error would lead to a recovered density roughly equal to the sum of the individual densities in the case of cylindrically symmetric filaments, and more ambiguous results in the case of asymmetric filaments. SMT measurements of the two-filament target and of each filament separately are shown in Fig. 4 . The left and right phase images in Fig. 4a each have bands with distinct slopes, confirming that the two plasmas are indeed located at different longitudinal positions. The middle phase image, which corresponds to the two-filament plasma, appears as a superposition of the other two phase images, with two separate bands at different angles. The presence of two independent filaments can thus be directly inferred from the phase images. 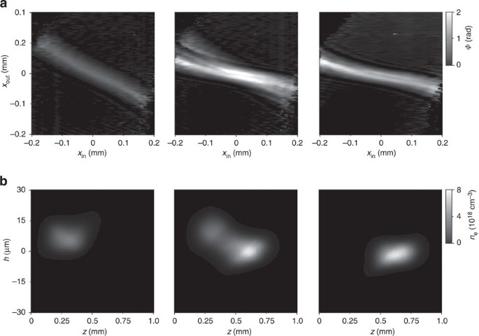Figure 4: Resolving the longitudinal structure of two plasma filaments. (a) Phase images for the upstream plasma only (left), both plasmas (middle) and downstream plasma only (right). (b) Electron density reconstructions for the phase images ina. Figure 4: Resolving the longitudinal structure of two plasma filaments. ( a ) Phase images for the upstream plasma only (left), both plasmas (middle) and downstream plasma only (right). ( b ) Electron density reconstructions for the phase images in a . Full size image The reconstructed electron-density profiles agree with the phase-image analysis above. The middle profile in Fig. 4b clearly shows a double-filament cross-section that is a superposition of the profiles on the right and left, confirming the ability of SMT to detect the hidden plasma filament in a single shot. To quantify the accuracy of this reconstruction, the filament longitudinal separation was measured using both a phase-band angle analysis (362 μm) and a density reconstruction analysis (360 μm). These values were then compared with an independent measurement using a burn-paper impression of the pump beams near focus (356±9 μm). All three values are very close to each other and show that SMT can resolve the plasma longitudinal position with better than 10 μm precision. A small transverse offset of about 14 μm between the two plasmas is also resolved and appears exaggerated by the disparity in the ranges of the horizontal and vertical axes of the density plots. Resolving ellipticity of filament cross-sections A more difficult test of the technique is the measurement of the cross-sectional structure of an individual plasma filament. Due to the astigmatism induced in the pump beams by detuning the angle of incidence on the focusing parabola, as described above, the LIPs generated were expected to be elliptical, making them ideal targets for this test. By making an assumption about the form of the cross-sectional profile, the degree of ellipticity and the orientation of the profile, as well as the limits on the longitudinal resolution of the technique, were obtained. We assumed a profile of the form: which describes a Gaussian profile with a peak density of n 0 and elliptic contours tilted by an angle φ with respect to the ( z , h ) coordinate system ( Fig. 5 ). The plasma was assumed to be located at the origin, without loss of generality. W || and W ⊥ correspond to the longitudinal and transverse 1/e-dimensions of the plasma, respectively, when φ= 0. The sinogram was then simulated by numerically integrating the phase shift accrued by rays passing through the profile as a function of angle, resulting in a band of phase similar to that in Fig. 2d . 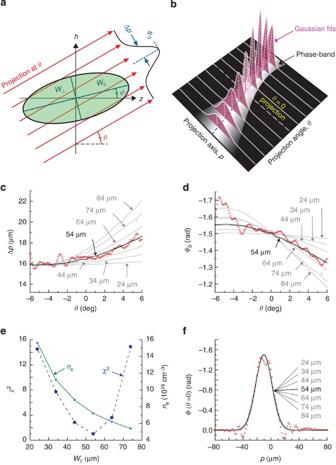Figure 5: Longitudinal resolution analysis for plasma 1. (a) Geometry of a projection of the elliptic density profile at angleθ. (b) Schematic depicting a sinogram (black and white intensity plot) and Gaussian fits (pink, semi-transparent curves shown in perspective) to the phase band line-outs for several angles. (c) Δp(θ) from the fits to the data (red circles) and to the models (black and grey curves). The black curve represents the best fit. (d)Φ0(θ) from the fits to the data (red circles) and to the models (black and grey curves). Note that the y axis is inverted to make interpretation more intuitive, as the refractive index of plasma is <1. (e)χ2analysis (blue, dashed line) of curves incnormalized to the best fit atW||=54 μm. Corresponding electron density (green, solid line) for each model. (f) Sinogram lineouts at 0 degrees for the data (red circles) and the models (black and grey curves). The model curves all overlap showing the insensitivity toW||. Note the invertedyaxis as ind. The simulated and measured sinograms were then compared by fitting the lineouts at each angle, θ , with a Gaussian of the form: Figure 5: Longitudinal resolution analysis for plasma 1. ( a ) Geometry of a projection of the elliptic density profile at angle θ . ( b ) Schematic depicting a sinogram (black and white intensity plot) and Gaussian fits (pink, semi-transparent curves shown in perspective) to the phase band line-outs for several angles. ( c ) Δ p ( θ ) from the fits to the data (red circles) and to the models (black and grey curves). The black curve represents the best fit. ( d ) Φ 0 ( θ ) from the fits to the data (red circles) and to the models (black and grey curves). Note that the y axis is inverted to make interpretation more intuitive, as the refractive index of plasma is <1. ( e ) χ 2 analysis (blue, dashed line) of curves in c normalized to the best fit at W || =54 μm. Corresponding electron density (green, solid line) for each model. ( f ) Sinogram lineouts at 0 degrees for the data (red circles) and the models (black and grey curves). The model curves all overlap showing the insensitivity to W || . Note the inverted y axis as in d . Full size image ( Fig. 5a,b ). The angular dependence of the fit parameters Φ 0 ( θ ) and Δ p ( θ ) was then used to constrain the model. For an elliptic profile, the projection, Φ ( p ), has the narrowest profile and the largest phase shift when the probing direction aligns with the major axis of the ellipse, that is, Δ p is minimized and Φ 0 is maximized when θ = φ . The fit data, Δ p ( θ ), could thus be used to determine φ , W ⊥ and W || , while Φ 0 (θ) was used to determine the density, n 0 . A normalized χ 2 analysis was performed on Δ p ( θ ), using W || as a parameter and keeping keeping Φ 0 (0) constant ( Fig. 5e ). The analysis yielded the following best-fit parameters: W || =54 μm, W ⊥ =16 μm, φ =6° and n 0 =7.2×10 18 cm −3 . The χ 2 curve shows that even a 10-μm deviation from the best fit is noticeable, indicating a density uncertainty of <18% ( Fig. 5d ). For comparison, the information available from a traditional single-projection diagnostic was extracted as a subset of the tomographic data corresponding to the 0-angle-of-incidence projection ( Fig. 5f ). The 0-angle lineouts show nearly equal agreement over the range of W || modelled, revealing the inability of this approach to resolve longitudinal structure. Making the traditional assumption of cylindrical symmetry resulted in an overestimate of the density by 300% for one plasma and 600% for the other. For the two-plasma target, the traditional diagnostic did not detect the presence of a second plasma, emphasizing the benefit of SMT. We have demonstrated that SMT can resolve the position and cross-sectional structure of an individual plasma filament, as well as detect the presence and position of multiple plasma filaments in a single-shot with high resolution. This capability has been a long-standing need within the laser–plasma community. Although the range of probing angles was limited to 12°, the technique was sensitive to positional and structural changes at the 10-μm level. In future work, these results can be improved upon and extended in many ways. For example, it is well within current technology to increase the range of probing angles to 60° or more, improving the resolving power by a factor of 5. Use of shorter wavelengths and more highly corrected optics also promise to provide significant improvements in resolution. Perhaps the most important factor, however, is the versatility and simplicity of this technique. The SMT concept can be implemented with probes spanning the full range of electromagnetic radiation, from radio waves to X-rays, and can also be used with non-electromagnetic sources such as ultrasound or electrons. It can be used in both phase-sensitive and amplitude-sensitive modes, allowing absorption-based as well as refractive-index-based studies. Alternatively, spectral multiplexing can be implemented in a mode where the angle of the rays is encoded by wavelength instead of the source position. This versatility of detection modalities allows SMT to be used in a very large range of applications. The ability to perform tomography with a single, broadband input beam is also a significant advantage, as many diagnostics involving single-beam probing of a target can be retrofitted to implement SMT by simply adding a grating and a lens to the probe line and using a spectrometer at the detection end. SMT also shows great promise as a way to perform through-wall imaging, which has long been of significant interest to the medical, defence and civilian fields [14] , [15] , [16] , [17] . A strongly scattering surface placed between an object and a detector normally prevents imaging of the object by randomizing the trajectory of probe rays emitted from or transmitting through the object. In SMT, however, the wavelength encoding of the rays allows unscrambling of the ray trajectories, provided the scattering surfaces are placed at either the focal plane or the object plane. SMT is thus ideally suited to the measurement of objects hidden behind or in-between walls that are transmissive, but highly scattering, opening up possibilities for an entirely new range of experiments involving ultrafast tomographic imaging. Laser system and pump beams Experiments were performed at the LOASIS program of the Lawrence Berkeley National Laboratory with a 1 kHz repetition-rate, 0.5 mJ, pulsed laser centred at 805 nm with a full-width-half-maximum bandwidth of 21 nm and a beam diameter of 5 mm. Beam splitters BS1 and BS2 ( Fig. 6a ) were used to create two nearly equal-intensity pump beams, each with separate delay lines, for generation of the LIPs. The two pumps were combined with a 0.4° angle onto an f =2″, 90° off-axis parabolic mirror, resulting in foci with significant astigmatism separated by 360 μm along the propagation direction of the probe. 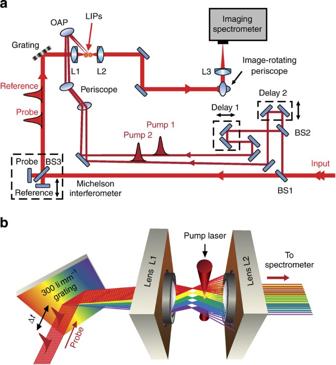Figure 6: Schematic of the experimental setup. (a) Layout of the experiment. A periscope and off-axis parabola (OAP), drawn in 3D perspective, were used to orient the focusing pumps normal to the measurement plane, which was parallel to the optical table. (b) Detail of the interaction showing how the spectral multiplexing was implemented. Only a single focusing pump laser is shown for clarity. Figure 6: Schematic of the experimental setup. ( a ) Layout of the experiment. A periscope and off-axis parabola (OAP), drawn in 3D perspective, were used to orient the focusing pumps normal to the measurement plane, which was parallel to the optical table. ( b ) Detail of the interaction showing how the spectral multiplexing was implemented. Only a single focusing pump laser is shown for clarity. Full size image Interferometry and phase detection The transmission of BS1 was sent to a Michelson interferometer to generate nearly identical reference and probe pulses, enabling acquisition of plasma-induced phase shifts by frequency domain interferometry [12] . The reference and probe pulses travelled along identical paths, but were timed so that the reference arrived before the creation of the plasma and the probe after. The two pulses interfered in the spectrometer, resulting in interferograms that recorded the phase difference between them as a function of wavelength and vertical position on the spectrometer slit. The phase difference was then correlated to the change in refractive index caused by the creation of the plasma. 'Null' shots taken without plasma were used to remove residual static background phase. Spectral multiplexing Position-encoded spectral multiplexing was achieved by using a 300 li mm −1 diffraction grating to generate angular dispersion, and an f =30 mm achromatic lens to convert the angular dispersion into a spatial dispersion of 15.6 μm nm −1 at the focus, providing a range of source positions spanning 430 μm ( Fig. 6b ). Each spectral component consisted of a cone of rays with an opening angle of 12°, however, only those rays lying within the measurement plane contributed to the measurement. The correlation between the source wavelength, λ, and the transverse position, x in , of the focus was determined by setting L to zero, so that the focal and object planes overlapped and the dispersed focus could be imaged by the spectrometer. The correlation between the vertical position y on the charge-coupled device to the output position x out was done by calibrating the magnification of the imaging system. The linear relationships between λ and x in and between y and x out allowed the raw interferometry data to be used for fast preliminary evaluation of the object, using the phase-image interpretation described above. Imaging and measurement-plane selection Achromatic lenses L2 and L3 and an image-rotating periscope were used to image a horizontal line 2.03 mm downstream of the focus, with a magnification of ×10 onto the vertical entrance slit of a 1/4 m imaging spectrometer with a 12-bit charge-coupled device camera ( Fig. 6 ). The slit, which was set to an opening of 80 μm, was used to select the specific cross-section of the plasma filaments measured (i.e., it was used to define the measurement plane shown in Fig. 1b ) by accepting only a subset of the transmitted probe rays. The measurement is thus necessarily averaged in the direction normal to the measurement plane over a distance equal to the slit width divided by the magnification, or roughly 8 μm. Generation of the sinogram The projection data, Φ ( p , θ ), known as a 'sinogram,' or a 'Radon transform' [18] , is obtained from the phase image by transforming to the ( p , θ ) coordinate system, which is related to the phase-image coordinates by: and ( Fig. 2a ). Transformation to the ( p , θ ) system was made considerably easier by first transforming to an intermediate coordinate system ( X , Y ), described by and , which is just a rotation by 45°. The remaining transformation can then be accomplished by two simple, 1D interpolations. For small angles, the Radon transform is related to the original spectral phase simply by a scale factor and a 45° rotation, making preliminary interpretation easy. Temporal resolution The temporal resolution of SMT is set by three time scales: the time required for probe rays to traverse the object, the range of arrival times of probe rays reaching the object and the coherence time of a source component. For the plasmas considered here, the first time scale was about 200 fs. The second consideration results from differences in the optical path-lengths of rays probing the measurement volume, which for millimeter-scale regions, is several picoseconds in general. Here, we measured a range in arrival times of 12 ps which was, in part, a result of setting up the measurement to allow longitudinal scanning of the plasma target. The third consideration comes from the fact that temporal modulations of the probe, caused by the interaction on timescales shorter than the coherence time, result in significant modulation of the source spectrum, distorting the spectral encoding. In these experiments, the optical bandwidth of an individual source component was about 0.2 nm, resulting in coherence lengths of about 2 ps. Although the temporal resolution achieved here was sufficient for characterizing the plasma filaments, which varied on a nanosecond timescale, optimization of the setup, by reducing the distance between the grating and lens L1, and by reducing the interaction volume should, in principle, improve the resolution to the 2–3 ps range. Further improvements could be made by using smaller target volumes and shorter wavelengths, with femtosecond resolutions achievable for micron-scale targets and X-ray probes. Longitudinal resolution The primary factors affecting the longitudinal resolution of SMT are the range of probing angles, the accuracy with which the ray trajectories can be discerned and the wavelength of the probing rays. The range of probing angles is set by the divergence of the source beams, which depends on the focusing geometry. The ability to measure the ray trajectories is affected by several factors, including the focal size of the spectral source components, which determines how well localized the source position x in is; the quality and resolving power of the imaging optics, which determines how well the ray output position x out can be measured; and the degree of diffraction and refraction experienced by the probe, which affects how well the ray picture of probe propagation applies to the interaction. For the ray picture of beam propagation to be valid, the Rayleigh range of the sources must be much smaller than L . To minimize diffraction effects, the object should be located at S out , and should be smaller in longitudinal extent than the depth of field of the imaging system. Shorter wavelength probes focus more tightly, experience less diffraction and refraction and generally behave more ray-like, permitting better resolution. In this work, an angular range of 12° was achieved. It is straight forward, however, and well within current technology to increase this range to roughly 60° by using f /1 focusing, potentially improving the resolution by a factor of 5. Achromatic doublets, which are only moderately well corrected for spherical and chromatic aberration, were used for both focusing and imaging of the rays. The toroidal imaging optics of the spectrometer, which have no chromatic aberration, but suffer significant astigmatism, also have a role in the overall image quality. Use of more highly corrected optics, which are readily commercially available, should thus also improve the resolution by another factor of a few. Despite the small range of angles, the results shown in Figs 3 and 5 indicate that the technique was sensitive to variations in both the longitudinal position and longitudinal structure at the 10 μm level or better. On the other hand, the plasma-density profile reconstructions, shown in Figs 2 and 4 , show resolutions on the order of 50 μm. This is due to a lack of optimization of the reconstruction algorithm implemented here, which was designed to demonstrate proof of principle. More sophisticated algorithms exist, and are the the topic of extensive research, which is beyond the scope of this work. How to cite this article: Matlis, N.H. et al . Single-shot ultrafast tomographic imaging by spectral multiplexing. Nat. Commun. 3:1111 doi: 10.1038/ncomms2120 (2012).